Translocation between PI(4,5)P2-poor and PI(4,5)P2-rich microdomains during store depletion determines STIM1 conformation and Orai1 gating The Orai1–STIM1 current undergoes slow Ca 2+ -dependent inactivation (SCDI) mediated by the binding of SARAF to STIM1. Here we report the use of SCDI by SARAF as a probe of the conformation and microdomain localization of the Orai1–STIM1 complex. We find that the interaction of STIM1 with Orai1 carboxyl terminus (C terminus) and the STIM1 K-domain are required for the interaction of SARAF with STIM1 and SCDI. STIM1–Orai1 must be in a PM/ER microdomain tethered by E-Syt1, stabilized by septin4 and enriched in PI(4,5)P 2 for STIM1–SARAF interaction. Targeting STIM1 to PI(4,5)P 2 -rich and -poor microdomains reveals that SARAF-dependent SCDI is observed only when STIM1–Orai1 are within the PI(4,5)P 2 -rich microdomain. Notably, store depletion results in transient localization of STIM1–Orai1 in the PI(4,5)P 2 -poor microdomain, which then translocates to the PI(4,5)P 2 -rich domain. These findings reveal the role of PM/ER tethers in the regulation of Orai1 function and a mode of regulation by PI(4,5)P 2 involving translocation between PI(4,5)P 2 microdomains. Ca 2+ is a unique second messenger whose cytoplasmic concentration is determined by Ca 2+ pumps and channels. Physiological receptor-evoked Ca 2+ signals regulate virtually all cell functions on timescales from ms to days [1] . At the same time, excess cytoplasmic Ca 2+ ([Ca 2+ ] i ) is highly toxic [2] , [3] . Most often, toxic [Ca 2+ ] i is due to excessive Ca 2+ influx through the plasma membrane (PM) Ca 2+ channels. Store-operated TRPC and Orai channels are key Ca 2+ influx channels [4] . While TRPC channels are mostly cell specific, all cells express the major isoform Orai1, which mediates the Ca 2+ release-activated Ca 2+ (CRAC) current [5] . Shortly after Orai1 is activated, it is partially inhibited by the rise in [Ca 2+ ] i : this limits Ca 2+ influx and prevents Ca 2+ toxicity [3] . Orai1 is activated in response to Ca 2+ release from the ER and is gated by the ER Ca 2+ sensor STIM1 (ref. 5 ). STIM1 has several domains including an ER-resident EF hand that mediates Ca 2+ sensing [6] ; a cytoplasmic coiled-coil domain 1 comprising an inhibitory helix that occludes STIM1 in the resting state [7] , [8] ; a SOAR domain that activates Orai1 (refs 9 , 10 ); a CTID domain that mediates interaction of the STIM1 inhibitor SARAF [11] with SOAR [12] ; a C terminus linker and a polybasic domain with multiple lysines (K-domain) that may mediate the interaction of STIM1 with PI(4,5)P 2 (ref. 13 ). Store depletion results in Orai1–STIM1 clustering in ER/PM microdomains. The nature of these domains and their role in Ca 2+ signalling is not well understood. Several recent studies have begun to define these domains. A search for proteins that tether the ER/PM in yeast [14] identified ER-resident homologues of mammalian extended synaptotagmins (E-Syts) [15] , VAP proteins, homologues of mammalian septins [16] and TMEM16 proteins. The three mammalian E-Syts participate in lipid transfer between the ER and PM [17] . Their role in ER/PM tethering depends on PM PI(4,5)P 2 and, in the case of E-Syt1, also on [Ca 2+ ] I (ref. 18 ). The E-Syts-formed tethers were suggested to be distinct from those formed by STIM1–Orai1 (ref. 18 ). However, the use of a PM/ER microdomain marker subsequently indicated that the receptor-evoked Ca 2+ signal forms E-Syt1-dependent tethers that recruit the phosphatidylinositol transfer protein Nir2; this restores PM PI(4,5)P 2 levels and sustains the Ca 2+ signal [19] . Finally, the filamentous septins 4 and 5 were reported to shape a PM PI(4,5)P 2 microdomain around clustered Orai1–STIM1 complexes [20] . However, the depletion of PI(4,5)P 2 does not inhibit the activation of Orai1 by STIM1 (ref. 21 ). Thus, the exact roles of PI(4,5)P 2 and the ER/PM microdomain in the regulation of Ca 2+ signalling and particularly Ca 2+ influx by Orai1 are not understood. A major regulatory modality of Orai1 is the inhibition by [Ca 2+ ] i to guard against excessive Ca 2+ influx. [Ca 2+ ] i inhibits Orai1 in two ways, fast Ca 2+ -dependent inactivation (FCDI) that occurs within 10–20 ms and slow Ca 2+ -dependent inactivation (SCDI) that develops in 1 min of channel activation [3] . SCDI (and possibly FCDI-see below) is mediated by the ER protein SARAF [11] , which interacts with STIM1 (ref. 12 ). In the present work, we use SCDI by SARAF as a reporter of the Orai1–STIM1 complex conformation and microdomain localization. We report that both STIM1–Orai1 complex formation and the STIM1 K-domain are required for the interaction of SARAF with STIM1. The STIM1–Orai1 complex must be present in a microdomain that is tethered by E-Syt1, which contains septin4, and that is enriched in PI(4,5)P 2 . Furthermore, SCDI is observed only when the STIM1–Orai1 complex is in a PI(4,5)P 2 -rich microdomain. Dynamics of the STIM1–Orai1 complex localization were measured by following fluorescence resonance energy transfer (FRET) between CFP-STIM1 and yellow fluorescent protein (YFP) targeted to the PI(4,5)P 2 -rich and -poor domains, revealing that the store depletion is followed by STIM1–Orai1 complex formation in the PI(4,5)P 2 -poor domain when the channel is fully active. This is in turn is followed by the translocation of the STIM1–Orai complex to the PI(4,5)P 2 -rich domain, recruitment of SARAF and SCDI. These findings identify a role for tethered ER/PM microdomains in regulating Ca 2+ influx and directing STIM1–Orai1 conformational changes, and report on a new mode of regulation by PI(4,5)P 2 . Orai1 C terminus facilitates interaction of SARAF with STIM1 Previous work reported that SARAF mediates the SCDI of Orai1 (ref. 11 ). Supplementary Fig. 1a shows that SARAF also affects FCDI. FCDI is affected by the STIM1:Orai1 ratio [22] , [23] . At a STIM1–Orai1 expression ratio of 1:1 and 20 mM EGTA in the pipette, (to minimize FCDI and better resolve the effect of SARAF), FCDI has mainly one component with a single time constant τ 1 of 7.0±0.5 ms ( n =3; in all results, the ± indicates s.e.m. and n indicates the number of experiments). In the presence of SARAF, FCDI is described best by two exponentials with time constants τ 1 of 15.4±0.2 and τ 2 of 241±26 ms ( n =3). The effect of SARAF on FCDI was not examined further in this study, as here we were interested mainly in using SCDI as readout of STIM1 conformation and localization in the PM/ER microdomain. Orai1 was reported to facilitate the interaction of SARAF with STIM1 (ref. 11 ). We extended these findings in Fig. 1a,b , which compare the time course of STIM1–STIM1, STIM1–Orai1 and STIM1–SARAF interaction using FRET ( Fig. 1a ) and co-immunoprecipitation (Co-IP; Fig. 1b ) assays. The basal FRET efficiency of STIM1–SARAF was somewhat higher than that of the basal FRET efficiency of STIM1–Orai1 and STIM1–STIM1 (see Supplementary Fig. 2a,b ). Therefore, to better illustrate the time course of FRET increase, Fig. 1a,c shows the normalized FRET ratio. The results show that the STIM1–SARAF interaction is increased minimally in the absence of Orai1. STIM1–STIM1 and STIM1–Orai1 FRET start shortly after the initiation of store depletion. Notably, FRET ( Fig. 1a ) and Co-IP ( Fig. 1b ) show that the STIM1–SARAF interaction is delayed by about 20–45 s. It then progresses more slowly than the STIM1–STIM1 and STIM1–Orai1 interactions. Several Orai1 mutants were used to identify the Orai1 domain that facilitates the STIM1–SARAF interaction ( Fig. 1c ). Orai1(Δ1–73), Orai1(ΔN) lacking the entire Orai1 amino terminus (N terminus), constitutively active Orai1(V102C) and channel-dead Orai1(R91W) facilitated the STIM1–SARAF interaction. Only Orai1(L273S) with a disrupted C terminus CCD [24] failed to support the STIM1–SARAF interaction. 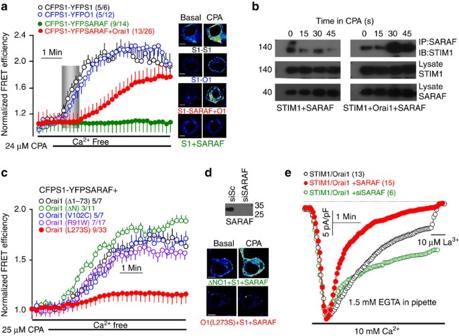Figure 1: STIM1–Orai1 interaction is required for SARAF interaction with STIM1. (a) FRET was measured in HEK293 cells transfected with CFP-STIM1 and YFP-STIM1, CFP-STIM1 and YFP-Orai1, CFP-STIM1 and YFP-SARAF and with (red) or without (green) HA-Orai1. Store depletion by CPA in Ca2+-free solution was initiated where indicated. The delay in STIM1–SARAF interaction is marked by grey rectangle. The averaged FRET efficiencies before and after 5 min treatment with CPA are shown inSupplementary Fig. 2. The images are example FRET images at the indicated conditions before (basal) and after 5 min store depletion. Scale bars, 5 μm. (b) Co-IP of STIM1 and SARAF. HEK cells were transfected with STIM1 and SARAF alone (left blots) or with Orai1 (right blots) and were incubated in Ca2+-free solution containing 25 μM CPA for the indicated times before preparation of lysates. The lysates were used to IP SARAF and blotted for STIM1. (c) CFP-STIM1-YFP-SARAF FRET was measured in cells expressing the indicated HA-Orai1 mutants. Scale bars in images are 5 μm. (d) HEK cells were treated with siSARAF for 48 h and analysed for expression of SARAF. (e) HEK cells were treated with scrambled or siSARAF were transfected with Orai1, STIM1 and with or without SARAF and Orai1 current was measured by dialyzing cells with pipette solution containing 1.5mM EGTA for 3 min in Ca2+-free bath. CRAC current was initiated by superfusing with a solution containing 10 mM Ca2+. The residual current was inhibited with 10 μM La3+. The same protocol was used in all current measurements unless otherwise stated. The currents were leak subtracted and normalized to the zero current to facilitate demonstrating the SCDI. Pick current density in pA/pF is given in the text. For all FRET experiments, of the two numbers listed in parenthesis next to the traces, the first indicates the number of experiments and the second indicates the number of cell analysed. All results (FRET and current) are given as the mean±s.e.m. Figure 1e shows the Orai1-mediated CRAC current. The current is activated by depleting ER Ca 2+ by including relatively low concentration (1.5 mM) of the slow Ca 2+ buffer EGTA in the pipette solution so that SCDI can be reliably measured. Three minutes after the initiation of store depletion, the current was measured by including 10 mM Ca 2+ in the bath solution. SARAF overexpression enhanced and its knockdown (see Fig. 1d ) markedly reduced SCDI. Figure 1: STIM1–Orai1 interaction is required for SARAF interaction with STIM1. ( a ) FRET was measured in HEK293 cells transfected with CFP-STIM1 and YFP-STIM1, CFP-STIM1 and YFP-Orai1, CFP-STIM1 and YFP-SARAF and with (red) or without (green) HA-Orai1. Store depletion by CPA in Ca 2+ -free solution was initiated where indicated. The delay in STIM1–SARAF interaction is marked by grey rectangle. The averaged FRET efficiencies before and after 5 min treatment with CPA are shown in Supplementary Fig. 2 . The images are example FRET images at the indicated conditions before (basal) and after 5 min store depletion. Scale bars, 5 μm. ( b ) Co-IP of STIM1 and SARAF. HEK cells were transfected with STIM1 and SARAF alone (left blots) or with Orai1 (right blots) and were incubated in Ca 2+ -free solution containing 25 μM CPA for the indicated times before preparation of lysates. The lysates were used to IP SARAF and blotted for STIM1. ( c ) CFP-STIM1-YFP-SARAF FRET was measured in cells expressing the indicated HA-Orai1 mutants. Scale bars in images are 5 μm. ( d ) HEK cells were treated with siSARAF for 48 h and analysed for expression of SARAF. ( e ) HEK cells were treated with scrambled or siSARAF were transfected with Orai1, STIM1 and with or without SARAF and Orai1 current was measured by dialyzing cells with pipette solution containing 1.5mM EGTA for 3 min in Ca 2+ -free bath. CRAC current was initiated by superfusing with a solution containing 10 mM Ca 2+ . The residual current was inhibited with 10 μM La 3+ . The same protocol was used in all current measurements unless otherwise stated. The currents were leak subtracted and normalized to the zero current to facilitate demonstrating the SCDI. Pick current density in pA/pF is given in the text. For all FRET experiments, of the two numbers listed in parenthesis next to the traces, the first indicates the number of experiments and the second indicates the number of cell analysed. All results (FRET and current) are given as the mean±s.e.m. Full size image These findings suggest that the STIM1–SARAF interaction is independent of the Orai1 channel function and can take place at basal [Ca 2+ ] i and that the interaction of STIM1 with the Orai1 C terminus CCD mediates recruitment of SARAF to the STIM1–Orai1 complex. Recruitment of SARAF to the complex starts only after initiation of the interaction between STIM1 and Orai1. The STIM1 K-domain in STIM1–SARAF interaction To determine if STIM1 domains other than SOAR are required for its interaction with SARAF, we tested the role of the STIM1 K-domain. Deletion of the K-domain prevented STIM1-SARAF interaction. This was the case even before store depletion as evident from the reduced basal FRET efficiency. This was not due to the interrupted STIM1–STIM1 or STIM1–Orai1 interaction ( Supplementary Fig. 1b ). Importantly, while deletion of the K-domain had no effect on the activation of Orai1 current by STIM1 (peak currents 19.1±0.5 and 18.8±0.5 pA/pF; n =4 and 6), the deletion eliminated the effect of SARAF on SCDI ( Fig. 2b ). 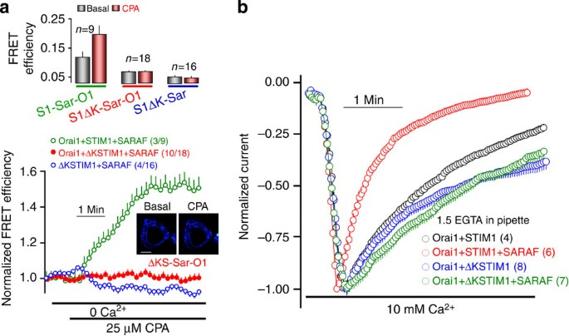Figure 2: SCDI by SARAF required the STIM1 K-domain. (a) HEK293 cells were transfected with Orai1, CFP-STIM1 or CFP-STIM1ΔK and YFP-SARAF, and FRET was measured in response to store depletion by 25 μM CPA in Ca2+-free solution. The columns show FRET efficiency before (basal) and 5 min after treatment with CPA. FRET efficiencies of the same experiments were normalized to show the time course of FRET changes in response to CPA. The images are examples of FRET images measured in cells expressing STIM1ΔK, SARAF and Orai1 before and after 5 min treatment with CPA, as indicated. Scale bars, 5 μm. (b) The Orai1 current and SCDI were measured with STIM1 or STIM1ΔK and in the presence and absence of SARAF. Results are given as mean±s.e.m of the indicated number of experiments. Figure 2: SCDI by SARAF required the STIM1 K-domain. ( a ) HEK293 cells were transfected with Orai1, CFP-STIM1 or CFP-STIM1ΔK and YFP-SARAF, and FRET was measured in response to store depletion by 25 μM CPA in Ca 2+ -free solution. The columns show FRET efficiency before (basal) and 5 min after treatment with CPA. FRET efficiencies of the same experiments were normalized to show the time course of FRET changes in response to CPA. The images are examples of FRET images measured in cells expressing STIM1ΔK, SARAF and Orai1 before and after 5 min treatment with CPA, as indicated. Scale bars, 5 μm. ( b ) The Orai1 current and SCDI were measured with STIM1 or STIM1ΔK and in the presence and absence of SARAF. Results are given as mean±s.e.m of the indicated number of experiments. Full size image To define the PM microdomain that interacts with the K-domain, we first determined whether the scaffold protein caveolin was required for normal current density and for SARAF to mediate SCDI. The knockdown of caveolin ( Supplementary Fig. 3a ) had no effect on current density but eliminated both the STIM1–SARAF interaction and the effect of SARAF on SCDI ( Supplementary Fig. 3b,c ). Hence, the STIM1–Orai1 complex has the same current whether in a caveolin-containing domain or outside this domain. However, the complex can only recruit SARAF to mediate SCDI when it is within the caveolin-containing domain. Therefore, SCDI by SARAF can function as a probe to report the microdomain localization of the STIM1–Orai1 complex. Tethered PM/ER microdomain in STIM1–SARAF interaction It has been suggested that the K-domain interacts with PM PI(4,5)P 2 (ref. 13 ). Therefore, we tested the effect of depleting PM PI(4,5)P 2 with the FRB/FKBP12 rapamycin-activated system [21] . The scheme in Fig. 3a illustrates the experimental system for Figs 3 and 4 and Fig. 3b shows that the FRB/FKBP12 system efficiently depletes cellular PI(4,5)P 2 . Supplementary Fig. 2c shows that the depletion of PI(4,5)P 2 reduces the basal STIM1–SARAF interaction (reduced basal FRET efficiency). More important, Fig. 3c shows that the depletion of PI(4,5)P 2 strongly inhibits the STIM1–SARAF interaction in response to store depletion. Significantly, as reported previously [21] , PI(4,5)P 2 depletion had no effect on Orai1 peak current (19.8±0.04 and 20.0±0.6 pA/pF without and with PI(4,5)P 2 depletion; n =8 and 6), but prevented the effect of SARAF ( Fig. 3d ). 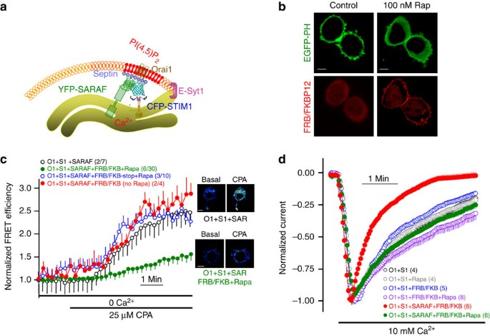Figure 3: SCDI by SARAF requires PM PI(4,5)P2. (a) A model illustrating a microdomain formed by PI(4,5)P2, tethered by E-Syt1 and stabilized by septins. (b) Cells transfected with EGFP-PH domain (green, PI(4,5)P2probe) and the FRB/FKBP12 (red, PI(4,5)P2depletion systems) were imaged before (left) and after exposure to 0.1 μM rapanycin for 2 min to deplete the PI(4,5)P2. Scale bars, 5 μm. (c) HEK293 cells were transfected with Orai1, STIM1 and SARAF and the FRB/FKBP12 or FRB/FKBP12-stop (no phosphatase control) and were either untreated (control) or treated with 0.1 μM rapamycin for 5 min to deplete PM PI(4,5)P2(red trace) and CFP-STIM1, YFP-SARAF FRET was measured in response to store depletion by 25 μM CPA in Ca2+-free solution. Basal and 5-min store depletion FRET efficiencies are shown inSupplementary Fig. 2. (d) Orai1 current was measured in cells transfected with Orai1, STIM1 and with or without SARAF and the FRB/FKBP12 system and SCDI by SARAF measured. Shown are rapamycin control (grey), FRB/FKBP12, no SARAF, no rapamycin control (blue) and FRB/FKBP12, SARAF, no rapamycin control (red). Depletion of PI(4,5)P2inhibited the effect of SARAF on SCDI (green). Results are given as mean±s.e.m of the number of experiments indicated in brackets. Figure 3: SCDI by SARAF requires PM PI(4,5)P 2 . ( a ) A model illustrating a microdomain formed by PI(4,5)P 2 , tethered by E-Syt1 and stabilized by septins. ( b ) Cells transfected with EGFP-PH domain (green, PI(4,5)P 2 probe) and the FRB/FKBP12 (red, PI(4,5)P 2 depletion systems) were imaged before (left) and after exposure to 0.1 μM rapanycin for 2 min to deplete the PI(4,5)P 2 . Scale bars, 5 μm. ( c ) HEK293 cells were transfected with Orai1, STIM1 and SARAF and the FRB/FKBP12 or FRB/FKBP12-stop (no phosphatase control) and were either untreated (control) or treated with 0.1 μM rapamycin for 5 min to deplete PM PI(4,5)P 2 (red trace) and CFP-STIM1, YFP-SARAF FRET was measured in response to store depletion by 25 μM CPA in Ca 2+ -free solution. Basal and 5-min store depletion FRET efficiencies are shown in Supplementary Fig. 2 . ( d ) Orai1 current was measured in cells transfected with Orai1, STIM1 and with or without SARAF and the FRB/FKBP12 system and SCDI by SARAF measured. Shown are rapamycin control (grey), FRB/FKBP12, no SARAF, no rapamycin control (blue) and FRB/FKBP12, SARAF, no rapamycin control (red). Depletion of PI(4,5)P 2 inhibited the effect of SARAF on SCDI (green). Results are given as mean±s.e.m of the number of experiments indicated in brackets. 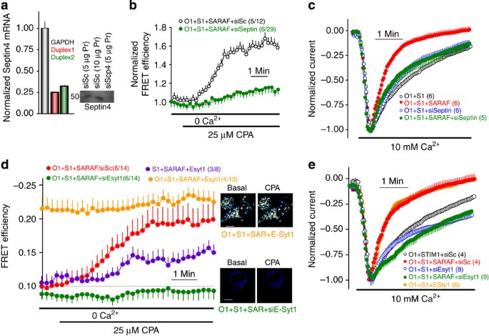Figure 4: SCDI by SARAF requires septin 4 and E-Syt1. (a) Effect of two siSeptin4 probes onseptin4mRNA measured by qPCR and effect of duplex 1 on septin4 protein. Lanes 1 and 3 were loaded with 5 μg protein and lane 2 with 10 μM protein. (b) CFP-STIM1/YFP-SARAF in the presence of Orai1 was measured in cells treated with scrambled or siSeptin4 in response to store depletion by 25 μM CPA in Ca2+-free solution. Basal and 5-min store depletion FRET efficiencies are shown inSupplementary Fig. 2. (c) Orai1 current was measured in cells expressing Orai1, STIM1 and with or without SARAF and treated with scrambled of siSeptin4. (d) FRET efficiency was measured in response to store depletion by 25 μM CPA in Ca2+-free solution in cells expressing CFP-STIM1, YFP-SARAF and E-Syt1 in the absence (purple) or the presence of Orai1 (orange) or cells treated with scrambled siRNA (red) or siE-Syt1 (green) and expressing Orai1, CFP-STIM1 and YFP-SARAF. Scale bars for all images are 5 μm. (e) The effect of E-Syt1 overexpression (orange) or knockdown (green) on SCDI by SARAF. Results are given as mean±s.e.m. of the number of experiments indicated in brackets. Full size image Figure 4: SCDI by SARAF requires septin 4 and E-Syt1. ( a ) Effect of two siSeptin4 probes on septin4 mRNA measured by qPCR and effect of duplex 1 on septin4 protein. Lanes 1 and 3 were loaded with 5 μg protein and lane 2 with 10 μM protein. ( b ) CFP-STIM1/YFP-SARAF in the presence of Orai1 was measured in cells treated with scrambled or siSeptin4 in response to store depletion by 25 μM CPA in Ca 2+ -free solution. Basal and 5-min store depletion FRET efficiencies are shown in Supplementary Fig. 2 . ( c ) Orai1 current was measured in cells expressing Orai1, STIM1 and with or without SARAF and treated with scrambled of siSeptin4. ( d ) FRET efficiency was measured in response to store depletion by 25 μM CPA in Ca 2+ -free solution in cells expressing CFP-STIM1, YFP-SARAF and E-Syt1 in the absence (purple) or the presence of Orai1 (orange) or cells treated with scrambled siRNA (red) or siE-Syt1 (green) and expressing Orai1, CFP-STIM1 and YFP-SARAF. Scale bars for all images are 5 μm. ( e ) The effect of E-Syt1 overexpression (orange) or knockdown (green) on SCDI by SARAF. Results are given as mean±s.e.m. of the number of experiments indicated in brackets. Full size image It has recently been reported that filamentous septin4 participates in the formation of a PI(4,5)P 2 microdomain around Orai1 and it is required for STIM1–Orai1 clustering and Orai1 activation [20] . We confirmed that the knockdown of septin4 ( Fig. 4a ) reduced Orai1 current by 36±3%. It is unlikely that this can be attributed solely to the disruption of a PI(4,5)P 2 microdomain [20] , since depletion of PI(4,5)P 2 did not reduce current density. Nevertheless, Fig. 4b,c and Supplementary Fig. 2d show that the knockdown of septin4 prevented STIM1–SARAF interaction and the effect of SARAF on SCDI (the currents were normalized to better demonstrate the effect of septin4 knockdown). Recent studies have shown that all three E-Syts participate in tethering the PM to the ER [18] and that E-Syt1 in particular has a key role [14] , [18] , [19] . Here we tested the effects of knockdown and overexpression of E-Syt1 on STIM1–SARAF interaction and SCDI. Preliminary experiments showed that HEK cells express predominantly E-Syt1 and E-Syt2 ( Supplementary Fig. 4a ) and that the knockdown of E-Syt1 increased E-Syt2 mRNA levels ( Supplementary Fig. 4b ). Although E-Syt2 and E-Syt3 were shown to localize to the peripheral ER and participate in PM/ER tethering [18] , the knockdown of E-Syt2 and E-Syt3 had no effect on SARAF-mediated SCDI ( Supplementary Figs. 4c,d ). In contrast, Fig. 4d shows that the knockdown of E-Syt1 (see Supplementary Fig. 4c ) reduced basal STIM1–SARAF FRET efficiency. Conversely, the overexpression of E-Syt1 maximally increased STIM1–SARAF FRET efficiency and FRET efficiency did not increase further by store depletion. The overexpression of E-Syt1 was sufficient to significantly increase STIM1–SARAF FRET efficiency in the absence of Orai1. These findings, together with the findings that the overexpression of E-Syt1 markedly increases the number and size of the PM/ER microdomains [18] , indicate that E-Syt1 overexpression preassembles the Orai1–STIM1–SARAF complex and thus no further recruitment of SARAF is observed on store depletion. Accordingly, Fig. 4e shows that knockdown of E-Syt1 prevented the SARAF-mediated SCDI, while the overexpression of E-Syt1 maximized SCDI to the level observed by the overexpression of SARAF, without affecting current density (Control 18.1±0.5, siE-Syt1 18.5±0.2, E-Syt1 18.0±0.7 pA/pF; n =4, 8, 6, respectively). Together the findings in Figs 3 and 4 suggest that tethering of the ER to the PM by E-Syt1 forms a microdomain that requires filamentous septins, is rich in PI(4,5)P 2 and to which the STIM1–Orai1 complex is targeted to recruit SARAF. In addition, the findings with the knockdown of the various E-Syts suggest some specificity in PM/ER tethers. The tethers formed by E-Syt1 recruit and regulate the function of the Orai1–STIM1 complex, while the extensive tethers formed by E-Syt2 and E-Syt3 (ref. 18 ) do not. Targeting STIM1 to defined PM/ER sites and SCDI by SARAF To support the hypothesis that the STIM1–Orai1 complex is targeted to the PI(4,5)P 2 -rich microdomain for interaction with SARAF, we sought means to target STIM1 to different PM microdomains. We achieved this using the Lyn- and Hras- or Kras-targeting motifs. These motifs were shown to target proteins to different PM microdomains [25] , [26] . The Kras and Hras motifs are fused to the C terminus, but the Lyn motif is commonly attached to the N terminus of proteins. However, since the STIM1 N terminus resides in the ER lumen, we fused all motifs to the C terminus of STIM1, which resulted in STIM1 targeting to the PM using all motifs, including STIM1-Lyn and STIM1-Hras. We determined their localization to test the specificity of the targeting. Supplementary Fig. 5a–c shows that STIM1-Kras and STIM1-Lyn are clustered in PM puncta in the absence of Ca 2+ store depletion. Importantly, the puncta formed by STIM1-Kras and STIM1-Lyn are likely not localized in the same microdomain. First, PM localization of STIM1-Lyn was eliminated by deletion of the STIM1 K-domain, while STIM1-Kras was retained in the PM puncta in spite of deletion of the K-domain ( Supplementary Fig. 6c,e ). Second, STIM1-Kras strongly co-IP’ed with SARAF, the Co-IP is independent of store depletion and it is not further enhanced by Orai1 ( Fig. 5d ). On the other hand, STIM1-Lyn does not Co-IP with SARAF regardless of the presence or absence of Orai1 or of store depletion ( Fig. 5d ). It was not possible to show the differential localization of STIM1-Kras and STIM1-Lyn in the same cells since the strong targeting motifs of STIM1-Kras and STIM1-Lyn recruited the respective STIM1s to the same puncta. This is illustrated in Supplementary Fig. 5d,e showing that STIM1-Kras and STIM1-Lyn recruited wild-type STIM1 to the same puncta. Nevertheless, the differential role of the K-domain and interaction with SARAF indicate that STIM1-Kras and STIM1-Lyn are targeted to different PM microdomains. 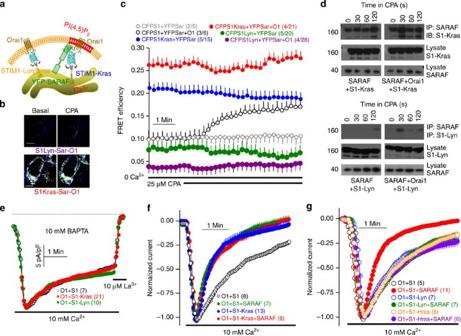Figure 5: Targeting STIM1 to PI(4,5)P2-poor and PI(4,5)P2-rich PM microdomains. (a) Scheme illustrating the microdomain targeting of STIM1 by the Lyn/Hras- and Kras-targeting motifs. (b) Examples of FRET images before and after treatment with CPA for 5 min in cells transfected with CFP-STIM1-Lyn+SARAF+Orai1 or STIM1-Kras+SARAF+Orai1 related to the experiments inc. Scale bars, 5 μm. (c) HEK293 cells were transfected with CFP-STIM1 and YFP-SARAF in the absence (grey) and presence of Orai1 (black); YFP-SARAF and CFP-STIM1-Kras (blue) or CFP-STIM1-Lyn (green) in the absence or presence of Orai1 (red and purple, respectively) and FRET efficiency was measured in response to store depletion by 25 μM CPA in Ca2+-free solution. (d) For the Co-IP, HEK cells were transfected with SARAF and either STIM1-Kras (upper blots) or STIM1-Lyn (lower blots) and with (right blots) or without Orai1 (left blots). The cells in Ca2+-free solution were treated with 25 μM CPA for the indicated times and were used to measure the Co-IP of STIM1 and SARAF. (e) Orai1 current was measured in pipette solution containing 10 mM BAPTA and bath containing 10 mM Ca2+to evaluate the spontaneous channel activity with STIM1 (black), STIM1-Kras (red) and STIM1-Lyn (green). In several experiments at each condition, where indicated, the residual currents were inhibited by 10 μM La3+. (f) SCDI was measured in pipette solution containing 1.5 mM EGTA and cells transfected with Orai1 and STIM1 (black, green), Orai1 and STIM1-Kras (blue, red) and in the presence of SARAF (red, green). (g) Experiments and conditions as inf, except that STIM1-Lyn or STIM1-Hras replaced STIM1-Kras. All results are given as mean±s.e.m of the number of experiments indicated in brackets. Figure 5: Targeting STIM1 to PI(4,5)P 2 -poor and PI(4,5)P 2 -rich PM microdomains. ( a ) Scheme illustrating the microdomain targeting of STIM1 by the Lyn/Hras- and Kras-targeting motifs. ( b ) Examples of FRET images before and after treatment with CPA for 5 min in cells transfected with CFP-STIM1-Lyn+SARAF+Orai1 or STIM1-Kras+SARAF+Orai1 related to the experiments in c . Scale bars, 5 μm. ( c ) HEK293 cells were transfected with CFP-STIM1 and YFP-SARAF in the absence (grey) and presence of Orai1 (black); YFP-SARAF and CFP-STIM1-Kras (blue) or CFP-STIM1-Lyn (green) in the absence or presence of Orai1 (red and purple, respectively) and FRET efficiency was measured in response to store depletion by 25 μM CPA in Ca 2+ -free solution. ( d ) For the Co-IP, HEK cells were transfected with SARAF and either STIM1-Kras (upper blots) or STIM1-Lyn (lower blots) and with (right blots) or without Orai1 (left blots). The cells in Ca 2+ -free solution were treated with 25 μM CPA for the indicated times and were used to measure the Co-IP of STIM1 and SARAF. ( e ) Orai1 current was measured in pipette solution containing 10 mM BAPTA and bath containing 10 mM Ca 2+ to evaluate the spontaneous channel activity with STIM1 (black), STIM1-Kras (red) and STIM1-Lyn (green). In several experiments at each condition, where indicated, the residual currents were inhibited by 10 μM La 3+ . ( f ) SCDI was measured in pipette solution containing 1.5 mM EGTA and cells transfected with Orai1 and STIM1 (black, green), Orai1 and STIM1-Kras (blue, red) and in the presence of SARAF (red, green). ( g ) Experiments and conditions as in f , except that STIM1-Lyn or STIM1-Hras replaced STIM1-Kras. All results are given as mean±s.e.m of the number of experiments indicated in brackets. Full size image The STIM1-Kras and STIM1-Lyn probes were then used to measure the FRET efficiency with SARAF under various conditions. Figure 5a illustrates the experimental protocol. As expected from the Co-IP results ( Fig. 5d ), STIM1-Lyn failed to recruit SARAF ( Fig. 5b,c ) when the two were co-expressed. Co-expression of Orai1 slightly reduced the basal STIM1-Lyn/SARAF FRET efficiency before and after Ca 2+ store depletion. Similarly, Supplementary Fig. 7 shows that the Hras motif also targets STIM1 to PM puncta in the absence of Ca 2+ store depletion and that STIM1-Hras failed to interact with SARAF. In sharp contrast, STIM1-Kras/SARAF displayed high FRET efficiency, which was maximized by the expression of Orai1 and did not increase by store depletion ( Fig. 5c ). Hence, the Kras motif targets STIM1 to a domain where it can recruit SARAF, whereas the Lyn and Hras motifs target STIM1 to a domain that prevents the recruitment of SARAF, although STIM1 can access Orai1 in both domains. The functional significance of targeting STIM1 to the different domains is shown in Fig. 5e–g . Figure 5e shows the CRAC current measured in the presence of the strong and fast Ca 2+ buffer 10 mM BAPTA to minimize SCDI and Supplementary Fig. 3d shows the Ca 2+ permeability of cells expressing STIM1-Kras alone. Notably, STIM1-Kras/Orai1 was largely constitutively active independent of store depletion, while STIM1-Lyn/Orai1 was not, although both generated puncta in the absence of store depletion ( Supplementary Fig. 5 ). However, the store depletion fully activated STIM1-Lyn/Orai1 and STIM1-Hras/Orai1 with similar current density to STIM1-Kras/Orai1 (19.7±0.9, 17.8±0.4 and 18.7±0.4 pA/pF, respectively; n =7, 5, 13, respectively). Most significantly, Fig. 5f,g show that the Orai1 current activated by STIM1-Kras undergoes rapid and strong SCDI with no further effect of SARAF, whereas the currents activated by STIM1-Lyn and STIM1-Hras are not affected by SARAF. The effects of targeting STIM1 by the Kras, Hras and Lyn motifs were not non-specific effects of extension of the STIM1 C terminus. Extending STIM1 C terminus by a similar size α helix had no effect on current amplitude (19.1±0.5 pA/pF; n =4) or SCDI by SARAF ( Supplementary Fig. 8 ). The results in Supplementary Figs 5–7 and Fig. 5 suggest that the Kras, Hras and Lyn motifs target STIM1 to different PM microdomains. STIM1-Kras is likely targeted to the domain dependent on caveolin/PI(4,5)P 2 /E-Syt1/septins, while STIM1-Lyn and STIM1-Hras are targeted to a different domain. STIM1-Kras and STIM1-Lyn/Hras then recruit Orai1 to the two respective domains. STIM1-Kras/Orai1, but not STIM1-Lyn-Hras/Orai1, then recruits SARAF to mediate SCDI. In support of this conclusion, the fast and maximal SCDI observed with STIM1-Kras is eliminated by the knockdown of SARAF ( Fig. 6a ), knockdown of caveolin ( Supplementary Fig. 3c ), depletion of PI(4,5)P 2 ( Fig. 6b ) and knockdown of E-Syt1 ( Fig. 6c ), while the SCDI observed with STIM1-Lyn is not affected by the depletion of PI(4,5)P 2 ( Fig. 6d ). 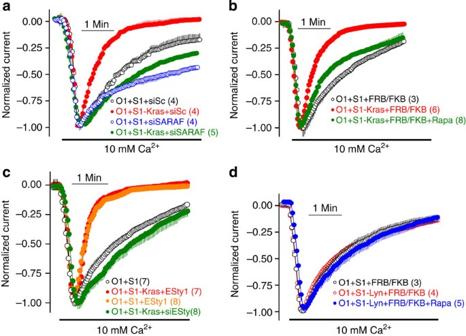Figure 6: The rate and maximal SCDI with STIM1-Kras requires native SARAF and intact PI(4,5)P2-rich microdomain. (a) Cells were treated with scrambled (black, red) or siSARAF (blue, green), and SCDI by STIM1 (black, blue) or STIM1-Kras (red, green) was measured. (b) SCDI by STIM1-Kras was measured in cells transfected with Orai1 and FRB/FKBP12 (red, control) and treated with rapamycin to deplete PI(4,5)P2(green). (c) SCDI by STIM1-Kras was measured in cells transfected with Orai1 and E-Syt1 (red) or treated with siE-Syt1 (green). The control orange trace is reproduced fromFig. 4e. (d) Depletion of PI(4,5)P2has no effect on the current measured with STIM1-Lyn (blue). Results are given as mean±s.e.m. of the number of experiments indicated in brackets. Figure 6: The rate and maximal SCDI with STIM1-Kras requires native SARAF and intact PI(4,5)P 2 -rich microdomain. ( a ) Cells were treated with scrambled (black, red) or siSARAF (blue, green), and SCDI by STIM1 (black, blue) or STIM1-Kras (red, green) was measured. ( b ) SCDI by STIM1-Kras was measured in cells transfected with Orai1 and FRB/FKBP12 (red, control) and treated with rapamycin to deplete PI(4,5)P 2 (green). ( c ) SCDI by STIM1-Kras was measured in cells transfected with Orai1 and E-Syt1 (red) or treated with siE-Syt1 (green). The control orange trace is reproduced from Fig. 4e . ( d ) Depletion of PI(4,5)P 2 has no effect on the current measured with STIM1-Lyn (blue). Results are given as mean±s.e.m. of the number of experiments indicated in brackets. Full size image Translocation of STIM1 between PI(4,5)P 2 microdomains The above findings indicate that the STIM1–Orai1 complex must localize to the PI(4,5)P 2 -rich domain to assume a conformation that allows it to recruit SARAF and mediate SCDI. Conversely, when the STIM1–Orai1 complex is in a PI(4,5)P 2 -poor domain it is in a conformation that cannot access SARAF, and thus the Orai1 current is more sustained. A critical question is whether STIM1 translocates between the two domains during physiological activation of the current. The first evidence that this is the case can be deduced from the delayed interaction between STIM1 and SARAF ( Fig. 1a,b ). Direct evidence for the shift of STIM1–Orai1 between microdomains is given in Fig. 7 . We targeted EGFP with N terminus Lyn motif or YFP with C terminus Hras motif to the PI(4,5)P 2 -poor domain and YFP with C terminus Kras motif to the PI(4,5)P 2 -rich domain ( Fig. 7a and model in Fig. 7b ). The probes were co-expressed with CFP-STIM1, and FRET in response to store depletion was measured. Most notably, FRET between Lyn-EGFP ( Fig. 7c ) or YFP-Hras ( Fig. 7d ) and CFP-STIM1 started upon start of store depletion but was transient and returned to basal levels within 1–2 min. Conversely, FRET between YFP-Kras and CFP-STIM1 started after a delay of about 1 min and then remained stable. Most notably, the depletion of PI(4,5)P 2 resulted in retention of STIM1 in the Lyn/Hras PI(4,5)P 2 -poor domain and its exclusion from the Kras PI(4,5)P 2 -rich domain. 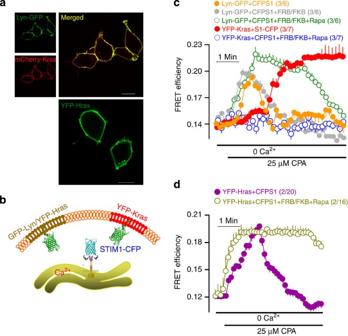Figure 7: Dynamic translocation of STIM1 between PI(4,5)P2-poor and PI(4,5)P2-rick domains in response to Ca2+store depletion. (a) PM localization of Lyn-GFP, mCherry-Kras and YFP-Hras. YFP-Kras shows similar PM localization. Scale bars, 5 μm. (b) The scheme illustrates the localization of Lyn-GFP/YFP-Hras and YFP-Kras. (c) HEK293 cells were transfected with CFP-STIM1, Lyn-GFP (orange, grey, green) or YFP-Kras (red, blue) and the PI(4,5)P2-depletion system (grey, green, blue) and were treated with 0.2 μM rapamycin (green, blue) or left untreated (grey, control). (d) The cells were transfected with CFP-STIM1 and YFP-Hras (purple) and the PI(4,5)P2-depletion system (dark yellow), and FRET was measured in response to store depletion by 25 μM CPA in Ca2+-free solution. Note the early but transient FRET with Lyn-GFP and YFP-Hras, the delayed but sustained FRET with YFP-Kras and the effect of PI (4,5)P2depletion on the two responses. Results are given as mean±s.e.m. of the number of experiments and cells indicated in brackets. Figure 7: Dynamic translocation of STIM1 between PI(4,5)P 2 -poor and PI(4,5)P 2 -rick domains in response to Ca 2+ store depletion. ( a ) PM localization of Lyn-GFP, mCherry-Kras and YFP-Hras. YFP-Kras shows similar PM localization. Scale bars, 5 μm. ( b ) The scheme illustrates the localization of Lyn-GFP/YFP-Hras and YFP-Kras. ( c ) HEK293 cells were transfected with CFP-STIM1, Lyn-GFP (orange, grey, green) or YFP-Kras (red, blue) and the PI(4,5)P 2 -depletion system (grey, green, blue) and were treated with 0.2 μM rapamycin (green, blue) or left untreated (grey, control). ( d ) The cells were transfected with CFP-STIM1 and YFP-Hras (purple) and the PI(4,5)P 2 -depletion system (dark yellow), and FRET was measured in response to store depletion by 25 μM CPA in Ca 2+ -free solution. Note the early but transient FRET with Lyn-GFP and YFP-Hras, the delayed but sustained FRET with YFP-Kras and the effect of PI (4,5)P 2 depletion on the two responses. Results are given as mean±s.e.m. of the number of experiments and cells indicated in brackets. Full size image Excess Ca 2+ influx is associated with, and in many cases is the initiator of, cellular and tissue pathologies. Hence, Ca 2+ influx channels are extensively regulated, most prominently by Ca 2+ itself, to restrict Ca 2+ influx. This is very well described for the Orai1 channel, which undergoes both FCDI and SCDI [3] , with STIM1 (refs 12 , 27 , 28 , 29 ) and SARAF ( Fig. 1 and Supplementary Fig. 1a ) participating in both through the STIM1 CTID domain [12] . The present work indicates that the regulation of Orai1 by Ca 2+ depends on the localization of the Orai1–STIM1 complex to specific PM microdomains and dynamic translocation of the complex between the microdomains; this sets the STIM1 conformation that recognizes SARAF. The microdomain is assembled by the E-Syt1-mediated tethering of the ER to the PM and appears to require several proteins known to demarcate PM microdomains, such as caveolin and septins. Caveolin is a scaffolding protein that participates in the formation of caveolae and assembly of signalling complexes [30] . Septins are a family of small GTPases that polymerize into non-polarized filaments and interact with both microtubules and the actin cytoskeleton to restrict distribution of proteins and lipids in the PM [31] . We note that the depletion of caveolin, E-Syt1 and PI(4,5)P 2 did not reduce the Orai1 current but only eliminated the effect of SARAF on SCDI. However, the depletion of septin4 while eliminated the effect of SARAF, also reduced the Orai1 current by about 36%. This would suggest that septins have a more global role in determining the composition and shape of the PM. A puzzling observation in the present study is that STIM1-Lyn and STIM1-Hras clustered at the PM but did not cause store-independent activation of Orai1, although the store depletion fully activated Orai1. Previous studies already concluded that STIM1 clustering is not sufficient to activate Orai1 (refs 10 , 12 ). However, in these cases, the STIM1 mutants were able to cluster but not activate Orai1, whereas STIM1-Lyn and STIM1-Hras fully activate Orai1. Moreover, when PI(4,5)P 2 is depleted, STIM1-Lyn is retained in the PI(4,5)P 2 -poor domain ( Fig. 7 ) and remains fully active. Together these findings suggest that the store depletion does more than co-clustering STIM1–Orai1 to activate the channel. This may be due to the dissociation of SARAF from STIM1, or due to the stabilization of a particular STIM1–Orai1 conformation. The present studies reveal dynamic translocation of the STIM1–Orai1 complex between PI(4,5)P 2 -poor and PI(4,5)P 2 -rich microdomains to control Ca 2+ influx. This is a new form of regulation by PI(4,5)P 2 that has not been previously described. Prior modes of regulation by PI(4,5)P 2 , including the regulation of ion transporters, has been attributed to a reduction or increase in PM PI(4,5)P 2 levels or to targeting of proteins to PI(4,5)P 2 -rich microdomains (reviewed in ref. 32 ). Dynamic translocation between PM microdomains with different PI(4,5)P 2 levels allows efficient temporal and spatial regulation independent of PI(4,5)P 2 synthesis and breakdown. Translocation back and forth between PI(4,5)P 2 microdomains should result in oscillatory activity of the regulated proteins. In the case of Orai1–STIM1, this will result in oscillations in Ca 2+ influx to support receptor-evoked Ca 2+ oscillations. STIM1 and SARAF are localized in the ER and interact to some extent in the basal state with filled Ca 2+ stores, as indicated by their basal Co-IP [12] ( Fig. 1b ) and FRET efficiency ( Figs 4d and 5c and Supplementary Fig. 2 ). Moreover, SARAF stabilizes STIM1 in the basal conformation since the knockdown of SARAF resulted in the store-independent clustering of STIM1 and Ca 2+ influx [11] , [12] . Activation of Ca 2+ influx by store depletion needs to relieve the basal inhibition of STIM1 by SARAF leading to the formation of the STIM1–Orai1 complex. Ca 2+ influx should be sustained for some time before its reinhibition by SARAF. The present studies provide evidence to suggest that the STIM1–Orai1 complex is first targeted to a PI(4,5)P 2 -poor microdomain, where STIM1 is in a conformation that fully activates Orai1 but minimally interacts with SARAF to increase Orai1 activity. Subsequently, the STIM1–Orai1 complex translocates to a PI(4,5)P 2 -rich microdomain ( Fig. 7 ) formed by tethering the ER and PM by E-Syt1 ( Fig. 4 ). In this microdomain, STIM1 is now in a conformation that binds SARAF, which mediates the SCDI to limit Orai1 activity. This mechanism allows the precise and timed regulation of Ca 2+ influx between fully activated and partially inhibited Ca 2+ influx to guard against cell toxicity. Constructs and antibodies STIM1-YFP, HA-Orai1, mCherry-Orai1, the Orai1 mutants and SARAF clones have been previously described [9] , [12] . The FKBP12 and FRB constructs are described in ref. 21 ). CFP-STIM1, CFP-STIM1ΔK and Orai1-CFP were a kind gift from Dr Murali Prakriya [33] . E-Syt1 was a gift from Dr Jen Liou [19] and E-Syt1, E-Syt2 and E-Syt3 were a kind gift from Dr Pietro DeCamilli [18] . Primers were obtained from Integrated DNA Technologies. All mutations were generated using the QuikChange Lightning site-directed mutagenesis kit from Agilent Technologies. Primers used for cloning are listed in Supplementary Table 1 . Preparation of the SARAF-myc has been previously described [12] . SARAF-YFP was made by digesting out SARAF at MluI and HindIII sites and ligating into pCMVYFP plasmid. STIM1-Kras, STIM1-Lyn, STIM1-Hras and Random α-helix constructs were made by mutating the bases in frame 5 amino acids downstream of the STIM1 open reading frame in CFP-STIM1. In brief, CFP-STIM1 plasmid was amplified using the specified primers and the Quick change lightning kit from Agilent and then the backbone was digested using dpnI enzyme. The primer sequences are shown in Supplementary Table 1 : Kras-Lys Lys Lys Lys Lys Lys Ser Lys Thr Lys Cys Val Ile Met; Lyn-Arg Asn Met Gly Cys Ileu Ser Lys Ser Lys Arg Lys Asp; Hras-Gly Cys Met Ser Cys Lys Cys Val Leu Ser; α-helix-Ala Ala Leu Lys Leu Ile Glu Ala Leu Ala Trp Glu Leu Ala. pYFP-Kras was made by mutating the amino acids to the Kras motif 3 amino acids downstream from YFP open reading frame. YFP-Hras was made by mutating the Hras motif 5 amino acids downstream from YFP open reading frame. p3xflag-mCherry-Kras was made by mutating to the Kras sequence 5 amino acids downstream of the open reading frame of mCherry. Lyn-pEGFP (Cat #35958) and PLCΔ1 PH-EGFP (Cat #21179) were purchased from Addgene. Antibodies used at the present work are: polyclonal anti-GFP (Life Technologies, Cat # A11122) 1:1,000; monoclonal anti-myc (Cell Signaling Inc., Cat # 2276) 1:1,000; polyclonal anti-SARAF (Thermo Fisher Scientific, Cat # PIPA524237) 1:100; polyclonal anti-Cav-1 (Sigma, Cat # C449-200) 1:500; polyclonal anti-E-syt1 (Sigma, Cat # SAB1105095) 1:250 and polyclonal anti-Septin (Sigma, Cat # SAB2501449) 1:200. siRNA probes and RT–PCR The scrambled control and short interfering RNA (siRNA) duplex sequences for SARAF, SEPTIN4, E-syt1 and Caveolin-1 are listed in Supplementary Table 1 . The siRNA sequences for E-Syt2 and E-Syt3 were the same as those used before [18] . HEK293 cells were plated at 70–80% confluence and transfected using Lipofectamine 2000 with siRNA duplexes after 12 h (20–40 nM per well) in six-well plates in serum-free medium according to the manufacturer’s protocol. The medium was changed to serum-containing medium 6 h after adding the duplexes to the cells. The cells were harvested after 48 h. The cells were harvested after 48 h. RNA was extracted using the TRIZOL reagent and the mRNA levels were determined by quantitative PCR as described [34] . In brief, the isolated mRNA was reverse transcribed into cDNA by the iscript cDNA synthesis kit from Bio-Rad Laboratories. The primers for quantitative reverse transcriptase-PCR for SARAF , Septin4 , E-Syt1 , E-syt2 , E-syt3 and GAPDH were purchased from Applied Biosystems. The fold change in the transcript levels of the specified genes was calculated by normalizing the Ct values from control and siRNA-transfected cells (threshold values) to GAPDH. FRET measurements HEK293 cells were plated at low confluence on glass bottom dishes (MatTek Corporation) and transfected with ECFP (donor) and EYFP (acceptor) tagged constructs, for 12–16 h using Lipofectamine 2000 (Invitrogen) at 37 °C. FRET imaging was performed at 37 °C using a confocal system (FV1000; Olympus) equipped with UplanSApo × 60 oil immersion objective (NA 1.35; Olympus) at × 1 zoom. Images were acquired at 10-s intervals using the simplified two-cube method for sensitized emission [35] , [36] . To minimize photobleaching, low laser power (1–3%) was used. Image analysis was performed with NIH ImageJ software. Images were corrected for background fluorescence as necessary. FRET was determined on a pixel-by-pixel basis using a two-step FRET efficiency calculation protocol [37] . In brief, bleed-through components were removed by generating a corrected FRET image (Fc) according to the equation Fc=I DA − d I DD where I DA and I DD are the background-subtracted FRET and ECFP images, respectively. The microscope-specific bleed-through constants a and d were determined by measuring the bleed-through from cells expressing ECFP or EYFP alone. The derived values were d =I DA /I DD =0.061±0.0064 ( n =52 cells) and a =I DA /I AA =0.02±0.0015 ( n =46 cells). In the second step, the apparent FRET efficiency ( E app ) was calculated using the algorithm E app =Fc/(Fc+ G I DD ) where E app is the fraction of ECFP exhibiting FRET and G is a microscope-specific constant derived by measuring the increase in ECFP fluorescence following EYFP acceptor photobleaching with the intramolecular CFP–YFP construct YFP–OASF–CFP [7] , which was estimated to be 0.69±0.12 ( n =18 cells). Confocal imaging For confocal imaging, Hela cells plated at low confluence on glass bottom dishes were transfected with the indicated constructs for 8–12 h. The images were captured at room temperature with UplanSApo × 60 oil immersion objective (NA 1.35; Olympus) at × 4 zoom. Images were processed with Photoshop CS3 (Adobe). PI(4,5)P 2 depletion PM PI(4,5)P 2 was depleted using the FRB/FKBP system provided by Dr Tamas Balla (NIH) and described in refs 38 , 39 . In brief, the PM Lyn-targeting sequence was fused to the FRB domain of mTOR1. The wild-type or kinetic-dead 5′-phosphatase was fused to FKBP12, which was tagged with mRFP. The two constructs were co-expressed in the cells. On exposure of the cells to rapanycin, the FRB and the FKBP12 heterodimerize to recruit the phosphatase to the PM and hydrolyse PI(4,5)P 2 . Current measurements HEK293T cells were cultured in Dulbecco’s modified eagle’s medium and 10% fetal bovine serum. Lipofectamine 2000 (Invitrogen) was used for cDNA or siRNA transfection. Treatment with siRNAs was with 20–40 nM for 48 h and transfection with cDNA was for 24–36 h before start of current recording. On the day of experiment, transfected cells were released and replated on square coverslips in 35-mm petri dishes and incubated with culture media for at least 1 h to allow attachment to the coverslips. Expression pattern and levels of the various constructs were carefully monitored by fluorescence microscopy. Electrophysiological experiments were performed at 20–24 °C using the patch-clamp technique in the whole-cell recording configuration. For current measurements, voltage ramps of −100 to 100 mV were applied every 4 s from a holding potential of 0 mV. The current at −100 mV was used to calculate current density as pA/pF. To measure SCDI, the pipette solution contained 135 mM CsCl, 6 mM MgCl 2 , 2 mM MgATP, 1.2 mm EGTA and 10 mm HEPES, pH 7.2 (with CsOH). During SCDI recording, after establishing the whole-cell configuration, the cells were kept in Ca 2+ -free solution for 5 min to allow store depletion before exposing the cells to bath solution containing 10 mM Ca 2+ . The standard bath solution contained 130 mM NaCl, 5 mM KCl, 1 MgCl 2 and 10 mM HEPES with or without 10 mM CaCl 2 (pH 7.4 with NaOH). To measure the extent of spontaneous current, the current was recorded as above except that 10 mM BAPTA replaced the 1.5 mM EGTA. Membrane potentials were amplified with an Axopatch 200B (Axon Instruments, Foster, CA, USA). The currents were filtered at 5 kHz and displayed on computer monitor. Where indicated, the currents were normalized first by averaging multiple experiments and then normalizing to the peak current. Peak currents are given in the text. Results were analysed using the Clampfit programme (Axon Instruments) and all currents are given as mean±s.e.m. Ca 2+ measurement Cells attached to coverslips were loaded with Fura2 by 30 min incubation at 37 °C with 5 μM Fura2/AM in culture media. After dye washing, florescence was measured at 340 and 380 nm using a TILL system as detailed before [12] . Collected images were analysed using MetaFluor and the results are given as the 340/380 ratio. Western blot and Co-IP measurements HEK293T cells were transfected with STIM1, SARAF and with or without Orai1. After 24 h, the cells were washed once in Ca 2+ -free solution and treated with 25 μM CPA for 0, 15, 30 or 45 s and the reactions were stopped and lysates prepared by a rapid removal of media and attrition of 0.5 ml of lysis buffer. Lysates (100 μl) containing the same amount of protein were cleared by incubation with 50 μl of Protein G Sepharose beads. The cleared lysates were used to IP STIM1 with anti-myc (SARAF) antibodies by incubation with 1 μl anti-myc antibody overnight at 4 °C. The complexes were collected by addition of 50 μl of Protein G Sepharose beads and incubation for 4 h at 4 °C. The precipitates were analysed for STIM1 (anti-GFP, 1:1,000) and SARAF (anti-myc, 1:1,000). Uncropped blot images are shown in Supplementary Fig. 9 . How to cite this article: Maléth, J. et al. Translocation between PI(4,5)P 2 -poor and PI(4,5)P 2 -rich microdomains during store depletion determines STIM1 conformation and Orai1 gating. Nat. Commun. 5:5843 doi: 10.1038/ncomms6843 (2014).